Spherical hyperlens for two-dimensional sub-diffractional imaging at visible frequencies Hyperlenses have generated much interest recently, not only because of their intriguing physics but also for their ability to achieve sub-diffraction imaging in the far field in real time. All previous efforts have been limited to sub-wavelength confinement in one dimension only and at ultraviolet frequencies, hindering the use of hyperlenses in practical applications. Here, we report the first experimental demonstration of far-field imaging at a visible wavelength, with resolution beyond the diffraction limit in two lateral dimensions. The spherical hyperlens is designed with flat hyperbolic dispersion that supports wave propagation with very large spatial frequency and yet same phase speed. This allows us to resolve features down to 160 nm, much smaller than the diffraction limit at visible wavelengths, that is, 410 nm. The hyperlens can be integrated into conventional microscopes, expanding their capabilities beyond the diffraction limit and opening a new realm in real-time nanoscopic optical imaging. The resolution of conventional imaging systems is inherently restricted by the diffraction limit, wherein the spatial information of features smaller than one-half of the wavelength is evanescent and cannot be projected to the far field [1] , [2] . Although near-field scanning optical microscopy can surpass this limit by collecting the evanescent field in close proximity to the object [3] , [4] , the slow scanning speed and non-negligible near-field perturbation from the scanning tip prevent its application in real-time imaging and biological systems. A superlens [5] , following Pendry's proposal [6] , which projects the sub-diffraction-limited images at the near field of the lens, was the first step towards real-time sub-diffraction resolution imaging. The major breakthrough emerged with the concept of optical hyperlenses [7] , [8] , [9] , showing the first proof-of-principal for magnifying sub-diffraction-scale objects to the far field as propagating waves. Using alternating dielectric and metallic layers in a curved geometry, this metamaterial-based optical device achieves strong optical anisotropy that supports the propagation of waves with very large spatial frequency and, because of the cylindrical geometry, adiabatically compresses its lateral wave vector while the wave is propagating outward along the radial direction [7] , [10] . Consequently, the sub-diffraction details of the objects are magnified to be above the diffraction limit and can be transmitted to the far field. Since the first experimental demonstration of the cylindrical hyperlens in one dimension [9] , newly improved designs as well as fabrication techniques, such as the impedance-matched [11] , flat [12] , oblate [13] , [14] , aperiodic [15] and acoustic [16] hyperlenses, have been proposed in the framework of transformational optics [17] , [18] , [19] . Nevertheless, all the experimental demonstrations of hyperlenses so far were limited to one-dimensional magnification and ultraviolet (UV) wavelengths, whereas for any practical imaging applications it is critical to demonstrate two-dimensional imaging, with resolution below the diffraction limit in the visible spectrum. Here, we present the first spherical hyperlens for two-dimensional sub-diffraction-limited real-time imaging at visible frequencies without the need for optical scanning or image reconstruction. Transforming scattered evanescent waves into propagating waves, the hyperlens produces a magnified image at the far field, where it could be further processed by conventional optics. The visible wavelength operation with sub-diffraction resolution opens new avenues towards optical nanoscope and real-time biomolecular imaging in living cells. 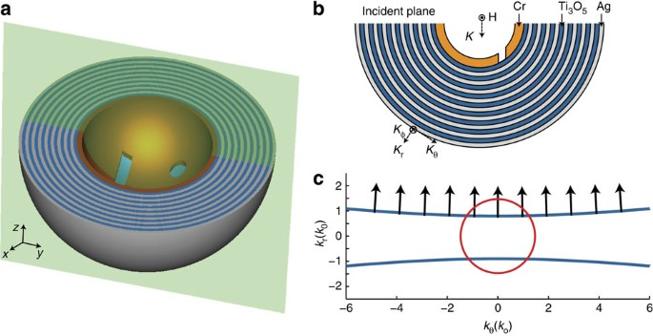Figure 1: Working principle of the spherical hyperlens. (a) Schematic of a spherical hyperlens comprised of nine pairs of silver and titanium oxide layers. (b) Cross section of the spherical hyperlens along the green incident plane. The object with sub-wavelength features is carved in a chromium layer atop the silver–titanium oxide multilayer (also shown in light blue ina). The transverse magnetic (TM) component of unpolarized light relative to the plane is labelled byK. (c) The isofrequency contour for the TM modes in the hyperlens compared with isotropic medium made of silicon oxide. The arrows, which are of unit length and on the ultraflat curve, show that all thekcomponents (including those much larger than the wave vectors available in dielectrics) propagate along the same radial direction, indicating the lack of diffraction. Design of the spherical hyperlens The spherical hyperlens is arranged in hemisphere geometry with alternating metallic and dielectric layers, as shown in Figure 1a with a cross section drawn in Figure 1b . When the thickness of each layer is much thinner than the wavelength of the incident light, the effective permittivity of the multilayer device can be described as the composite average, in the radial (normal to the metal-dielectric interfaces) direction and in the tangential direction (along the metal-dielectric interfaces). r̂ , θ̂ and follow the conventional definitions of the radial, polar and azimuth directions, respectively, in spherical coordinates, as shown in Figure 1b . A small-positive ɛ θ together with a large-negative ɛ r results in the propagation of a transverse magnetic wave being governed by a flat hyperbolic isofrequency contour shown in Figure 1c , which allows the propagation of waves with much larger spatial frequencies than in natural media. On the other hand, the transverse electric components, having no electric field along the radial direction, propagate through the hyperlens as a low-index isotropic medium such that the non-zero spatial frequencies are filtered out. Hence, the objects can only be magnified in one direction under linear polarized illumination. We overcome this restriction by illuminating the sample with unpolarized light, which contains transverse magnetic components spanning the whole two-dimensional reciprocal space, thus supporting propagation of sub-wavelength features in both dimensions. At the same time, the spherical geometry, along with the diffraction control enabled by the flat dispersion, result in a gradual magnification of the sub-wavelength objects during the radial transmission, wherein the evanescent waves are adiabatically transformed into the propagating waves. Consequently, a magnified image is formed at the output plane of the hyperlens, which can be subsequently acquired though a conventional optical microscope. Figure 1: Working principle of the spherical hyperlens. ( a ) Schematic of a spherical hyperlens comprised of nine pairs of silver and titanium oxide layers. ( b ) Cross section of the spherical hyperlens along the green incident plane. The object with sub-wavelength features is carved in a chromium layer atop the silver–titanium oxide multilayer (also shown in light blue in a ). The transverse magnetic (TM) component of unpolarized light relative to the plane is labelled by K . ( c ) The isofrequency contour for the TM modes in the hyperlens compared with isotropic medium made of silicon oxide. The arrows, which are of unit length and on the ultraflat curve, show that all the k components (including those much larger than the wave vectors available in dielectrics) propagate along the same radial direction, indicating the lack of diffraction. Full size image Material and fabrication constraints Visible wavelength operation requires a high-index dielectric material to match the magnitudes of permittivities in the metal and dielectric layers at the operation frequency [20] . Therefore, we choose titanium oxide to be the dielectric material with a dielectric constant of 5.83 at 410 nm, whereas the permittivity of silver at this wavelength is −4.99+0.22i [21] . The filling ratio is chosen to be 1:1, with a layer thickness of 30 nm. The ultimate resolution limit is set by the magnification as well as the thickness of each layer, below which the multilayer cannot be considered as an effective medium. Being <1/10 of the wavelength, the effective medium approximation is met, and the effective radial and tangential permittivities can be derived: ɛ r =−64−19.83i and ɛ θ =0.42−0.11i. The high contrast between the radial and tangential permittivities results in an ultraflat unbound dispersion relation over a large range of wave vectors, allowing the sub-wavelength information to propagate in the hyperlens. 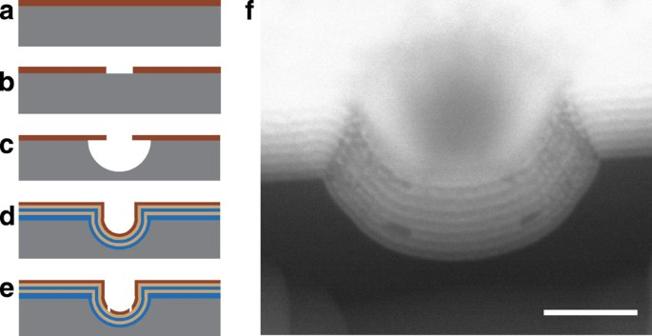Figure 2: Structure and fabrication procedure of the spherical hyperlens. (a) Chromium hard mask layer is deposited on a quartz wafer. (b) Opening window is made. (c) Isotropic wet etching defines a half-spherical geometry, and the mask layer is removed. (d) A total of 18 layers are conformally deposited onto the hyperlens structure. (e) Chromium layer is deposited to engrave arbitrary objects. (f) A scanning electron microscope image of the cross-sectional view of spherical hyperlens. The multilayer stack is clearly seen. Scale bar, 500 nm. The fabrication process is schematically shown in Figure 2a–e . Initially, the half-spherical geometry of the hyperlens is formed by isotropic wet etching into the quartz substrate. Nine pairs of silver and titanium oxide thin film layers were subsequently deposited, with a layer thickness of 30 nm. Finally, the arbitrary sub-diffraction-limited features are inscribed on an additional chromium layer by focused ion beam milling to serve as objects for imaging. The final structure is confirmed by cutting a cross section of the spherical hyperlens ( Fig. 2f ). Figure 2: Structure and fabrication procedure of the spherical hyperlens. ( a ) Chromium hard mask layer is deposited on a quartz wafer. ( b ) Opening window is made. ( c ) Isotropic wet etching defines a half-spherical geometry, and the mask layer is removed. ( d ) A total of 18 layers are conformally deposited onto the hyperlens structure. ( e ) Chromium layer is deposited to engrave arbitrary objects. ( f ) A scanning electron microscope image of the cross-sectional view of spherical hyperlens. The multilayer stack is clearly seen. Scale bar, 500 nm. Full size image Observation of resolution beyond the diffraction limit The hyperlens is placed in a transmission optical microscopy system such that it serves as an integral part of the microscope with the ability to deliver the sub-wavelength features into the propagation regime, where they can be collected by the objective lens. 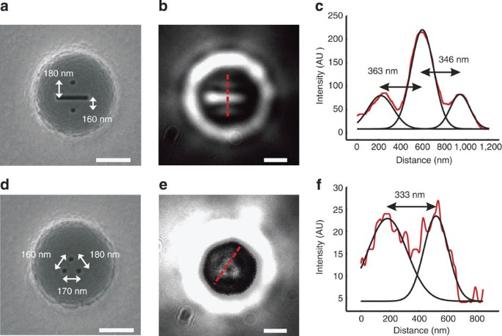Figure 3: Measurement with the magnifying hyperlens. (a) Scanning electron microscope (SEM) image of object 1: two 100 nm diameter dots separated by a 100 nm wide bar. The gap sizes are 180 and 160 nm. All scale bars shown in the figure are 500 nm. (b) Image taken of the object being magnified by the hyperlens. The sub-diffraction-limited objects were clearly resolved by the spherical hyperlens. Along the red dash line, a cross section is taken to calibrate the performance of the hyperlens. (c) Cross-sectional analysis showing separation by 363 and 346 nm, respectively, corresponding to ×2.1 magnification. (d) SEM image of object 2: three dots positioned triangularly with gaps of 180, 170 and 160 nm. (e,f) Image and cross section of the object along the red line after being magnified. Figure 3 depicts two sets of the magnified images of sub-diffraction-limited objects, obtained by CCD (charge-coupled device) camera at the image plane. The objects shown in Figure 3a consists of two apertures of 100 nm diameter and a slot of 100 nm width, which are separated by 160 and 180 nm, respectively. The magnified optical image on the hyperlens is shown in Figure 3b . The result indicates that the separation of 160 and 180 nm is clearly resolved in the experiment, despite being below the diffraction limit of the 410 nm illumination wavelength. Figure 3c presents the cross section along the red line in Figure 3b, showing a measured distance between dots and bars of 346 and 363 nm, corresponding to magnifications of 2.02–2.16. A different object, made of three apertures located in triangular configuration with 160, 170 and 180 nm spacing in three sides ( Fig. 3d ), is also clearly resolved at the far field ( Fig. 3e ); the separation of the two apertures is measured to be 333 nm in the cross-sectional analysis shown in Figure 3f . Given the fabricated distance of 160 nm, the averaged magnification ratio is 2.08. This ratio is smaller than the designed value, which is mainly because of non-conformal deposition and inaccurate thickness control of the layer, resulting in deviation of the concentricity of the hyperlens and a position-dependent magnification power. Figure 3: Measurement with the magnifying hyperlens. ( a ) Scanning electron microscope (SEM) image of object 1: two 100 nm diameter dots separated by a 100 nm wide bar. The gap sizes are 180 and 160 nm. All scale bars shown in the figure are 500 nm. ( b ) Image taken of the object being magnified by the hyperlens. The sub-diffraction-limited objects were clearly resolved by the spherical hyperlens. Along the red dash line, a cross section is taken to calibrate the performance of the hyperlens. ( c ) Cross-sectional analysis showing separation by 363 and 346 nm, respectively, corresponding to ×2.1 magnification. ( d ) SEM image of object 2: three dots positioned triangularly with gaps of 180, 170 and 160 nm. ( e , f ) Image and cross section of the object along the red line after being magnified. Full size image In addition, the hyperlens magnifies the image of the objects onto a spherical surface; the resulting distortions in subsequent conventional microscope image are shown in Figure 3b,d . Adapting thin-film deposition techniques with improved conformality, thickness and roughness control can considerably improve the quality of the hyperlens, and in principle, these image aberrations can be compensated by introducing more corrections conventionally employed in lens design. Full-wave three-dimensional simulation To further support our experimental results, we performed a full-wave three-dimensional electromagnetic simulation with Finite Element Analysis (COMSOL). The radii of the inner and outer spherical surfaces of the hyperlens are taken as 210 and 500 nm, respectively, making the designed magnification ratio 2.4. 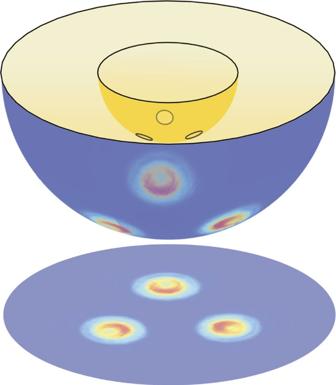Figure 4: Full-wave simulation of the working hyperlens. A finite element analysis shows the magnified image of sub-diffraction-limited objects. The objects are composed of three circular openings on perfect electric conductor. The diameter of each circle is 50 nm, and the distance between the circles is 150 nm. The working wavelength is 410 nm. At the image plane, the distance between the circles is |360 nm. Figure 4 shows the hyperlens imaging of three apertures with 150 nm separation inscribed on the inner surface. The electric field distribution at the outer spherical surface of the hyperlens clearly shows how the three apertures at the inner surface are magnified to three bright spots, with separation of 360 nm in good agreement with the analytical calculations, showing a magnification of 2.4 in both x - and y -directions. By increasing the ratio between the inner and outer radius of the hyperlens, the magnification and resolution can be further improved while reducing the transmission of the hyperlens. Figure 4: Full-wave simulation of the working hyperlens. A finite element analysis shows the magnified image of sub-diffraction-limited objects. The objects are composed of three circular openings on perfect electric conductor. The diameter of each circle is 50 nm, and the distance between the circles is 150 nm. The working wavelength is 410 nm. At the image plane, the distance between the circles is |360 nm. Full size image By implementing the principle of hyperbolic dispersion into the innovative spherical geometry, we have designed and demonstrated the first hyperlens that projects an optical image onto the far field, with resolution beyond the diffraction limit in both lateral directions on the object plane. Our results indicate that with real material and practical fabrication techniques, the hyperlens can be operated at the visible frequency, which is of vital importance to biological applications. Improved thin-film deposition techniques will eliminate the distortion found in the current experiments to a considerable extent. This spherical hyperlens can be readily integrated with optical microscopes, as the magnified images from the hyperlens are comprised of propagating waves, and can be further manipulated by conventional optics in real time. The unique sub-diffraction imaging capability and visible frequency operation of the presented hyperlens make it competent for next-generation optical metrology, molecular imaging and nanolithography. Sample fabrication As shown in Figure 2a–e , spherical hyperlens fabrication starts with a highly refined quartz wafer (Fused Silica Corning 7980 of UV Grade 1″ square × 0.006″±0.001″ thick, Corning). To prevent the pinholes made from deposition, at least 100-nm-thick chromium is necessary for the etching mask. Circular opening as small as 50 nm is followed by focused ion beam milling (Strata 201XP, FEI). The half-spherical geometry of the hyperlens is formed by isotropic wet etching into the quartz substrate with 10:1 buffered oxide etchant. The shape of the lens is defined by the etching mask, and the diameter is precisely controlled by the etching time. The spherical shape of the etched cavity is examined by atomic force microscope (Dimension 3100, Veeco). After removing chromium mask layer by another wet etching with CR-7 etchant, electron beam evaporation system (EB-4P, Torr) was used to deposit the silver and titanium oxide multilayer. To reduce the scattering from the surface roughness, vacuum condition is kept at 10 −7 Torr and the film growth rate is kept as slow as 0.1 nm s −1 . During the process, we calibrated the refractive index of different phases in titanium oxide, and found that titanium pentoxide (Ti 3 O 5 ) has a higher refractive index (2.42) at 410 nm, which is preferable to our experiment. As the last step, one additional layer of 50 nm chromium is deposited, and the arbitrary sub-diffraction-limited features such as nanometer-sized apertures and slots are inscribed by focused ion beam milling. The surface roughness of the final multilayer structure is <1.5 nm r.m.s. Experimental setup The experiment is operated in a normal transmission optical microscopy system, wherein the objects on the inner hyperlens surface are illuminated by a normally incident and unpolarized white light source (XE120, EXFO), with a 10 nm band pass filter centred at 410 nm. A magnified image on the outer surface is then imaged through the objective (×100 oil immersion objective, NA=1.3, Zeiss) and captured by EM-CCD camera (NS-H9100-02, Hamamatsu). Multiple exposures are taken and averaged to increase the signal-to-noise ratio. Simulation method The full-wave three-dimensional electromagnetic simulation ( Fig. 4 ) is performed in COMSOL. The hyperlens is represented by an effective medium with permittivity tensor (1) in the Cartesian coordinate: where ( r , θ , φ ) is the spherical coordinate triplet; meanwhile ɛ r , ɛ θ and ɛ φ are defined in the result section. The surrounding medium in Figure 4 is silicon oxide. The object at the inner surface is composed of three circular openings in a perfect electric conductor. The distance between the circles is 150 nm, which is smaller than the diffraction limit at 410 nm wavelength. In the simulation, the radial polarized illumination condition is applied to represent the unpolarized light used in the experiment. How to cite this article: Rho, J. et al . Spherical hyperlens for two-dimensional sub-diffractional imaging at visible frequencies. Nat. Commun. 1:143 doi: 10.1038/ncomms1148 (2010).